Enhanced second-harmonic generation from metal-integrated semiconductor nanowires via highly confined whispering gallery modes Coherent and tunable nanoscale light sources utilizing optical nonlinearities are required for applications ranging from imaging and bio-sensing to on-chip all-optical signal processing. However, owing to their small sizes, the efficiency of nanostructures even with high nonlinear coefficients is poor, therefore requiring very high excitation energies. Although surface-plasmon resonances of metal nanostructures can enhance surface nonlinear processes such as second-harmonic generation, they still suffer from low conversion efficiencies owing to their intrinsically low nonlinear coefficients. Here we show highly enhanced and directional second-harmonic generation from individual CdS nanowires integrated with silver nanocavities (>1,000 times higher external efficiency compared with bare CdS), in which the lowest-order whispering gallery mode is engineered to concentrate light in the nonlinear material while minimizing Ohmic losses. The directional nonlinear signal is redirected into another waveguide, which is then utilized to configure an optical router that can potentially serve as a tunable coherent light source to enable on-chip signal processing for integrated nanophotonic systems. Integrated nanophotonic systems [1] require the development of a large set of devices with functionalities ranging from light emission, directed transport, detection to modulation, switching and routing, with high efficiency and small footprints. Furthermore, it would be desirable if a single material system can demonstrate all these required functionalities, as it would enable seamless integration of these devices to assemble nanophotonic systems [2] . Recently, semiconductor nanowires (NWs) have been configured into a variety of nanophotonic devices including lasers [3] , waveguides [4] , photodetectors [5] , modulators and all-optical switches [6] , all from a single material, cadmium sulfide (CdS). Although CdS is not the only system that can provide these functionalities, it serves as a good test case to experiment the idea of obtaining integrated nanosystems from a single functional material. Another device element essential for optical circuits and other applications is a tunable source of coherent radiation, which can be obtained by utilizing the nonlinearities of the material to enable photon–photon interactions. In this nonlinear realm, second-harmonic generation (SHG), an important nonlinear process that converts an electromagnetic wave of frequency ω (fundamental wave, FW) into another wave with twice the frequency (2 ω ), has been demonstrated for ZnO, GaN, KNbO 3 , CdS, ZnTe and InP NWs [7] , [8] , [9] , [10] , [11] , [12] . However, these studies involved bare NWs with substantially low conversion efficiency (typically ~10 −9 W −1 ) owing to their small intrinsic size and poor field confinement and/or spatial overlap with the material [10] . The low efficiency of SHG in nanostructures implies that very high optical energies are required to produce nonlinear signals that can be utilized for any practical applications. Therefore, improving the efficiency of nonlinear signal generation from nanostructures with small interaction volumes but without compromising their small footprints is essential. A common strategy is to engineer optical cavities, which can strongly confine light to produce larger nonlinear signals. Whispering gallery mode (WGM) dielectric cavities, typically exhibiting high Q values but with much larger footprints, have been utilized to improve second-order nonlinear interactions [13] , [14] . Surface-plasmon resonances (SPRs) of metal nanostructures have been extensively studied to enhance surface nonlinear processes such as SHG [15] , [16] , [17] , [18] , [19] , [20] , [21] , but the nonlinear conversion efficiency is still extremely low owing to their intrinsically low nonlinear coefficients [22] . Hybrid systems, for example, nanoscale nonlinear dielectrics coupled to metallic structures, utilize the local-field enhancement of SPRs to enhance SHG, but suffer from high-Ohmic losses at the metal–dielectric interface, and poor spatial overlap with the nonlinear material [23] , and may not be used for waveguiding applications. For example, sub-100 nm dielectric nanoparticles coupled with plasmonic cavities have demonstrated large enhancements of the SHG signal based on SPRs [24] , in which the enhanced field on the surface can significantly overlap with the nonlinear dielectrics. However, for nanostructures such as NW with dimensions smaller than the wavelength of the incident light, WGMs are loosely confined and exhibit high loss [25] , and hence not very useful for nonlinear optical applications such as SHG. Furthermore, use of SPRs for the enhancement of the SHG signal for these intermediate sized particles (>150 nm) or NWs [23] may not be too efficient because of the lower overlap of the surface-plasmon modes with the bulk of the nonlinear material. Here, we report a hybrid metal–semiconductor nanostructure [23] , [26] , [27] , that is, a Ag-coated CdS NW, in which CdS has a large nonlinear coefficient of ~78 pm V −1 (>2 times larger than lithium niobate) [28] , to engineer highly confined lowest-order WGM, which is used to facilitate tunable, directional and efficient SHG output. We chose the diameter of CdS NWs in the >150-nm range in order to optimize the SHG signal output while also optimizing their waveguiding properties to enable their applications in nanophotonic circuitry. Effective concentration of light in the nonlinear region combined with a large nonlinear coefficient of CdS significantly enhances light–matter interaction in this device leading to >1,000 times enhancement of the SHG conversion efficiency (external), thus enabling it to be coupled into other functional devices at low excitation energies. Moreover, the directionality and the higher intensity of the SHG signal produced by NWs is utilized to configure an optical router, which can be useful for the design of functional nanophotonic systems. Characterization and mechanism of enhanced SHG from metal-coated NWs Experiments were performed on single-crystalline CdS NWs grown mostly along the c axis ( Supplementary Fig. 1 ) that were dispersed onto a glass substrate followed by the fabrication of the Ag cavity ( Fig. 1a ; see Methods section). In order to excite SHG, a tunable Ti:sapphire laser was focused onto individual devices through the glass substrate ( Fig. 1a ) with the electric field polarized along the c axis (transverse magnetic, TM; see Methods section and Supplementary Fig. 2 ). Room temperature measurements carried out on a Ag-coated CdS NW (diameter, d =230 nm) at 950 nm excitation yielded a bright blue spot at the excitation region ( Fig. 1b ). The emission spreads outwardly and symmetrically, and propagates perpendicular to the NW’s long axis ( Supplementary Fig. 3 ). We observed a sharp peak (4 nm full-width at half-maximum) at ~475 nm, that is, at twice the frequency of the FW at 950 nm, as expected for SHG ( Fig. 1c ). The normalized external SHG conversion efficiency, η 2 ω , is estimated to be ~3.0 × 10 −6 W −1 ( , where P ω ( P 2 ω ) represents the peak power of the FW (SHG); see Methods section) from the Ag-coated CdS NW, is ~300 times higher than that obtained from the same NW (~9.2 × 10 −9 W −1 ) before Ag deposition ( Fig. 1c ) and is much higher than other reported metal-related nanostructures (~10 −9 W −1 ; ref. 16 ). Another important metric, that is, SHG scattering cross-section ( σ 2 ω ), is ~3.1 × 10 8 GM from the Ag-coated device ( , 1 GM=10 −50 cm 4 s per photon; Supplementary Table 2 and Supplementary Discussion ). 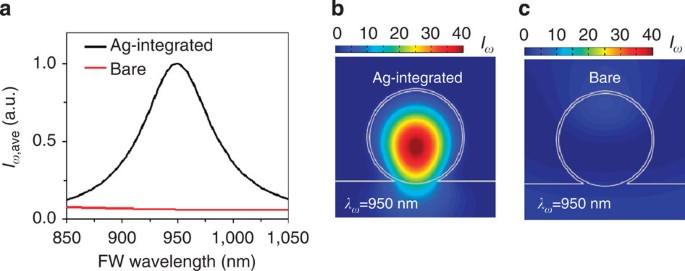Figure 2: Resonant modes supported in Ag-coated CdS nanowires (NWs) under transverse magnetic excitation. (a) Normalized average intensity (Iω,ave) of fundamental wave (FW)-excited modes in the nonlinear region of Ag-coated (black) and bare (red) NWs. (b,c) Calculated intensity distribution (Iω=|Eω|2) of the mode excited by the FW in Ag-coated (b) and bare (c) NWs (d=230 nm). The white lines depict the SiO2interlayer. For both Ag-coated and bare CdS NWs, photoluminescence (PL) resulting from two-photon absorption [11] , [12] is also observed near 502 nm. When we moved the excitation laser far away from the NWs and focused it on glass/Ag (background), there was no measurable SHG signal ( Fig. 1c ), while measurements performed on bare and Ag-coated Si NWs also did not show any observable SHG signal, which shows that the signal is produced from the active material, that is, CdS, but enhanced by the metal coating. Power-dependent measurements revealed a quadratic response to the excitation power ( Fig. 1d ), also characteristic of SHG. Furthermore, the SHG signal is predominantly TM polarized (that is, along the CdS c axis, Fig. 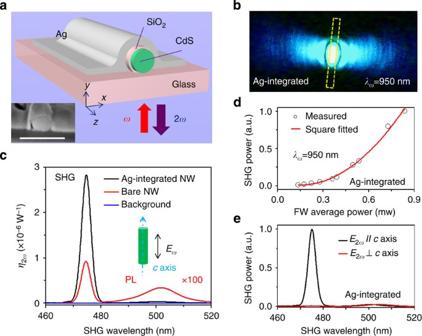1e ) under TM excitation, which is related to the largest second-order nonlinear coefficient of CdS along the c axis ( d 33 ; Supplementary Discussion ). Figure 1: Enhanced second harmonic generation (SHG) from Ag-coated CdS nanowire (NW) devices. (a) Schematic of a Ag-coated CdS NW with an Ω-shaped cross-section. The CdS core is the nonlinear region. Upon illumination from the glass side (ydirection) by the fundamental wave (FW;ω), back-scattered SHG (2ω) signal is collected. Inset: scanning electron microscope image of the cross-sectioned (by focused ion beam) device. Scale bar, 500 nm. (b) Real colour dark-field optical image of the SHG signal propagating perpendicular to the NW’s long axis obtained from a Ag-coated CdS NW device. The yellow dashed rectangle outlines the device. (c) Conversion efficiencyof SHG signal from Ag-coated (black) and the same bare (red, multiplied 100 × ) CdS NW (diameter,d=230 nm) along with the background (blue) signal. Inset: FW is tuned atλω=950 nm with transverse magnetic (TM; the electric filed polarized along thecaxis) polarization. (d) SHG power response as a function of the excitation (average) power, which fits to a square dependence. (e) Polarization properties of the SHG signal under parallel (FW) excitation obtained for the same Ag-coated CdS NW device. Figure 1: Enhanced second harmonic generation (SHG) from Ag-coated CdS nanowire (NW) devices. ( a ) Schematic of a Ag-coated CdS NW with an Ω-shaped cross-section. The CdS core is the nonlinear region. Upon illumination from the glass side ( y direction) by the fundamental wave (FW; ω ), back-scattered SHG (2 ω ) signal is collected. Inset: scanning electron microscope image of the cross-sectioned (by focused ion beam) device. Scale bar, 500 nm. ( b ) Real colour dark-field optical image of the SHG signal propagating perpendicular to the NW’s long axis obtained from a Ag-coated CdS NW device. The yellow dashed rectangle outlines the device. ( c ) Conversion efficiency of SHG signal from Ag-coated (black) and the same bare (red, multiplied 100 × ) CdS NW (diameter, d =230 nm) along with the background (blue) signal. Inset: FW is tuned at λ ω =950 nm with transverse magnetic (TM; the electric filed polarized along the c axis) polarization. ( d ) SHG power response as a function of the excitation (average) power, which fits to a square dependence. ( e ) Polarization properties of the SHG signal under parallel (FW) excitation obtained for the same Ag-coated CdS NW device. Full size image To explore the underlying mechanism of TM-excited SHG enhancement, we used a two-dimensional model to calculate the average intensity ( I ω ,ave ) of the modes excited by FW in Ag-coated and bare NWs (see Methods section and Supplementary Equation (8) ). As shown in Fig. 2a , the Ag cavity markedly alters the optical response of the device in the FW spectral range [26] . A strong resonant peak for the Ag-coated NW ( d =230 nm) at ~950 nm is observed, whereas there is no such feature in the same spectral range for the bare NW ( Supplementary Fig. 4a ). At the resonant wavelength of the Ag-coated NW, the optical mode is highly concentrated in the core of the device ( Fig. 2b ) in contrast to the bare NW ( Fig. 2c ). Therefore, the thick Ag deposition serves as an efficient mirror to keep the light from leaking out, therefore forming a highly confined WGM nanocavity [29] . The mode profile corresponds to the fundamental mode, TM 01 (refs 30 , 31 , 32 ), which is the lowest-order WGM, and owing to the metal coating exhibits a much better field confinement in comparison with bare dielectric NWs [29] , [32] . Therefore, the average intensity of the mode is enhanced inside the Ag-coated CdS NW in comparison with the bare NW ( Fig. 2a and Supplementary Fig. 5e ), which noting ( Supplementary Equation (7) ) leads to the enhancement of the observed SHG signal ( Fig. 1c ). Moreover, the mode profile in the Ag-coated NW ( Fig. 2b and Supplementary Fig. 6a ) has negligible spatial overlap between the optical fields and Ag or CdS surfaces, suggesting that symmetry breaking from these interfaces are minimally involved in the SHG process, which is also in agreement with the data ( Fig. 1c ). Figure 2: Resonant modes supported in Ag-coated CdS nanowires (NWs) under transverse magnetic excitation. ( a ) Normalized average intensity ( I ω ,ave ) of fundamental wave (FW)-excited modes in the nonlinear region of Ag-coated (black) and bare (red) NWs. ( b , c ) Calculated intensity distribution ( I ω =| E ω | 2 ) of the mode excited by the FW in Ag-coated ( b ) and bare ( c ) NWs ( d =230 nm). The white lines depict the SiO 2 interlayer. Full size image Size- and excitation polarization dependence of the SHG signals In order to understand the effect of NW size on the SHG signal generated under TM excitation, we plot the calculated average intensity of the optical mode confined in the CdS region as a function of (excitation) wavelength and CdS NW diameter in Fig. 3a . It can be seen that the resonant wavelength redshifts with increasing diameter of the CdS NW, which also suggests the tunability of the SHG response with NW size. Size- and wavelength-dependent measurements ( Fig. 3b , data shown for three Ag-coated CdS NWs with d =220, 230 and 240 nm) performed on various NWs exhibit maximum SHG signals at different excitation wavelengths ( Supplementary Fig. 7a ), which is in agreement with the calculated signal intensities (see Methods section and Supplementary Equation (7) ). The enhancement of SHG is observed to be >1,000 × in the Ag-coated CdS device in comparison with the bare NW ( d ~240 nm; Fig. 3c and Supplementary Fig. 7b ). For larger CdS NW devices, for example, d =360 nm, the TM 01 mode redshifts away from our experimentally accessible spectral range; however, another mode, TM 11 , moves into this spectral range ( Supplementary Fig. 8 ), thereby leading to resonance-enhanced but still TM-polarized SHG. 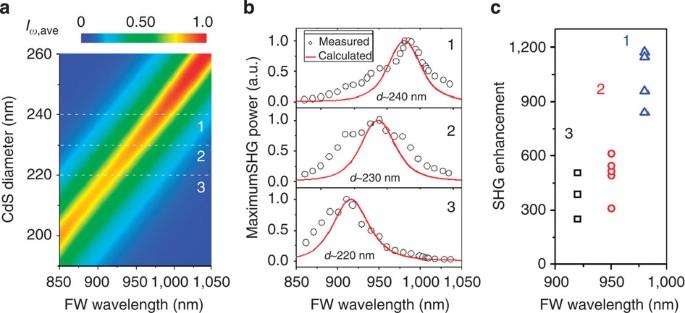Figure 3: Size-dependent properties of transverse magnetic (TM)-excited second harmonic generation (SHG) in Ag-coated CdS nanowires (NWs). (a) Two-dimensional plot of normalizedIω,aveas a function of FW wavelength and CdS diameter. The dashed white lines labelled 1, 2 and 3 correspond to the CdS diameter values,d=240, 230 and 220 nm, respectively. (b) Measured and calculated SHG signal power as a function of FW wavelength in three Ag-coated NW devices (CdS diameter, 240, 230 and 220 nm). Here we assume(Supplementary Equation (7)) and the number 1 (or 2, 3) is associated with the relevant dashed line ina. (c) SHG enhancement obtained for Ag-coated NW devices in comparison with the bare NWs (d=240 (1), 230 (2) and 220 nm (3)). Enhancement of >1,000 × is observed ford~240 nm Ag-CdS NWs over bare CdS. Figure 3: Size-dependent properties of transverse magnetic (TM)-excited second harmonic generation (SHG) in Ag-coated CdS nanowires (NWs). ( a ) Two-dimensional plot of normalized I ω ,ave as a function of FW wavelength and CdS diameter. The dashed white lines labelled 1, 2 and 3 correspond to the CdS diameter values, d =240, 230 and 220 nm, respectively. ( b ) Measured and calculated SHG signal power as a function of FW wavelength in three Ag-coated NW devices (CdS diameter, 240, 230 and 220 nm). Here we assume ( Supplementary Equation (7) ) and the number 1 (or 2, 3) is associated with the relevant dashed line in a . ( c ) SHG enhancement obtained for Ag-coated NW devices in comparison with the bare NWs ( d =240 (1), 230 (2) and 220 nm (3)). Enhancement of >1,000 × is observed for d ~240 nm Ag-CdS NWs over bare CdS. Full size image In order to study the polarization anisotropy of SHG from the Ag-coated CdS NW ( d =230 nm), we rotate the polarization angle ( θ ) of the FW from 0° (corresponding to the NW’s c axis, TM mode) to 90° (perpendicular to the NW’s c axis, transverse electric (TE) mode) gradually, and observed that the SHG signal decreases monotonically in excellent agreement with theoretical calculations at 950 nm excitation ( Fig. 4a and Supplementary Equation (2) ). The main reason for the angle dependence of SHG signal on FW polarization is that TM excitation can couple into NWs more efficiently than the TE polarization [33] . If the transverse SPR mode is excited under TE excitation ( θ =90°), SHG can also be generated, but it is not as efficient in comparison with TM excitation (discussed latter). Under TE excitation, the wavelength-dependent SHG performed on the Ag-coated device ( d =230 nm) exhibits a peak ~980 nm (a transverse SPR mode) and is in excellent agreement with theory ( Fig. 4b and Supplementary Equation (7) ). The TE-excited SHG signal at 980 nm corresponds to a conversion efficiency of ~4.0 × 10 −8 W −1 ( Fig. 4c ) and is ~40 times higher in comparison with the same bare NW. This enhancement is because the field confinement (owing to the transverse SPR) in the Ag-coated NW ( Fig. 4d ) is much stronger (>10 × ) than the bare NW ( Fig. 4e ). Moreover, the TE-excited SHG signal is still polarized along the CdS c axis ( Supplementary Equation (1) and Supplementary Fig. 9b ). 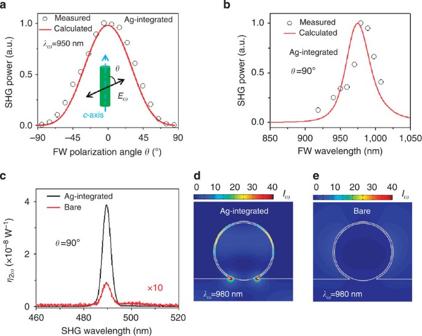Figure 4: Polarization dependent second harmonic generation (SHG) in a 230-nm diameter Ag-coated CdS nanowire (NW). (a) Polarization dependence of SHG at 950 nm excitation. Inset: FW polarization angleθis set with respect to the CdScaxis (also growth axis). (b) Measured and calculated wavelength dependence of SHG under TE excitation (θ=90°) (Supplementary Equation (7)). (c) Conversion efficiency of TE-excited SHG signal collected from Ag-coated (black) and bare (red, multiplied 10 × ) NWs excited at 980 nm. (d,e) Calculated intensity distribution of FW-excited modes in Ag-coated (d) and bare (e) NWs excited at 980 nm. Similar tob, FW is TE polarized inc–e. Figure 4: Polarization dependent second harmonic generation (SHG) in a 230-nm diameter Ag-coated CdS nanowire (NW). ( a ) Polarization dependence of SHG at 950 nm excitation. Inset: FW polarization angle θ is set with respect to the CdS c axis (also growth axis). ( b ) Measured and calculated wavelength dependence of SHG under TE excitation ( θ =90°) ( Supplementary Equation (7) ). ( c ) Conversion efficiency of TE-excited SHG signal collected from Ag-coated (black) and bare (red, multiplied 10 × ) NWs excited at 980 nm. ( d , e ) Calculated intensity distribution of FW-excited modes in Ag-coated ( d ) and bare ( e ) NWs excited at 980 nm. Similar to b , FW is TE polarized in c – e . Full size image Coupling of SHG signals from a device into another on-chip waveguide The utility of nanoscale on-chip coherent light sources is enhanced if the output light can be coupled into other functional devices. This idea was demonstrated by redirecting or coupling the SHG signal from a Ag-coated CdS NW into another CdS waveguide [4] . In our experiments, we investigated T-type structures (NWs not touching at the junction) that were found randomly when NWs were dry-transferred ( Fig. 5a ). In a T-type structure with two NWs, one NW was optically excited to produce the SHG signal (source NW, S-NW) while the other was utilized as a waveguide (waveguide NW, W-NW). The excitation laser was tuned at 1,020 nm (to produce SHG at 510 nm, which is below the band gap of CdS) [4] and was focused at a reference point (R), slightly away from the T-junction. Strong SHG was observed to symmetrically radiate outwards ( Fig. 5b,c ) from the excitation region (similar to Fig. 1b ). However, when we move the excitation laser at the junction (J), the SHG spot was observed to be very bright but asymmetric ( Fig. 5d,e ); one of the SHG branches was completely redirected and launched into the W-NW, which propagates along the W-NW to finally exit from the other end ( Fig. 5e ). The coupling between S-NW and W-NW seems to be very efficient, which also benefits from the directionality of the SHG signal. The theoretical calculation shows that >50% of the SHG signal can be confined in the NW waveguide ( Supplementary Discussion ). Notice that FW may also be scattered directly into the W-NW owing to the edge scattering effect and then produce the SHG signal as it propagates in the W-NW. However, the W-NW is observed to produce much weaker SHG than S-NW when directly illuminated. Moreover, this edge effect is highly polarization dependent; the excitation (FW) polarized perpendicular to the edge of the W-NW results in weak FW scattered/coupled into the structure in comparison with parallel excitation (to the edge) ( Supplementary Fig. 10a,b ), and therefore gives rise to poor SHG output at the other end ( Supplementary Fig. 10c,d ). Therefore, the direct scattering of the FW into the W-NW can be ruled out based on the conversion efficiency (of W-NW) and polarization argument. The other possibility of the excitation laser directly exciting the W-NW can also be ruled out as the SHG signal should have propagated orthogonal to the NW’s long axis (similar to Fig.1b and Supplementary Fig. 11 ), contrary to what is observed ( Fig. 5e ). Therefore, the SHG signal excited at the T-junction of the S-NW is efficiently coupled into the W-NW and waveguided to the end ( Fig. 5f,g ) and demonstrates that the coherent SHG signals can be routed into other devices. 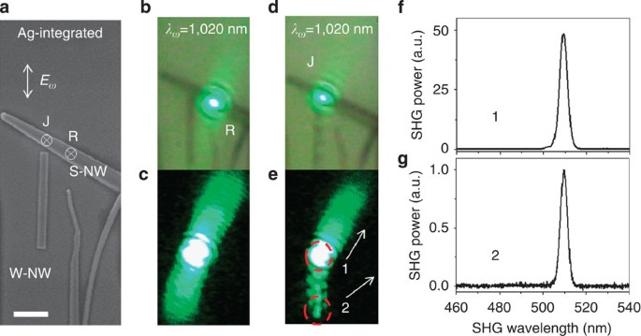Figure 5: Redirecting second harmonic generation (SHG) from a Ag-coated CdS nanowire (NW) (S-NW) to another NW (W-NW). (a) Scanning electron microscope image of a T-type structure formed by S-NW and W-NW. The excitation is polarized along the long axis of W-NW. J (R) stands for the junction (reference point) on the S-NW. Scale bar, 2 μm. (b,c) Optical image of symmetrical SHG signal emanating from the reference point (R) of S-NW in the bright (b) and dark (c) field mode. (d,e) SHG from the junction (J) of S-NW launched into W-NW in the bright (d) and dark (e) field mode. Here label 1 (or 2) represents the junction (or output port of W-NW). (f,g) SHG signal collected from 1 (f) and 2 (g). The data from 1 is normalized by the maximum of that obtained from 2. Figure 5: Redirecting second harmonic generation (SHG) from a Ag-coated CdS nanowire (NW) (S-NW) to another NW (W-NW). ( a ) Scanning electron microscope image of a T-type structure formed by S-NW and W-NW. The excitation is polarized along the long axis of W-NW. J (R) stands for the junction (reference point) on the S-NW. Scale bar, 2 μm. ( b , c ) Optical image of symmetrical SHG signal emanating from the reference point (R) of S-NW in the bright ( b ) and dark ( c ) field mode. ( d , e ) SHG from the junction (J) of S-NW launched into W-NW in the bright ( d ) and dark ( e ) field mode. Here label 1 (or 2) represents the junction (or output port of W-NW). ( f , g ) SHG signal collected from 1 ( f ) and 2 ( g ). The data from 1 is normalized by the maximum of that obtained from 2. Full size image Configuration and characterization of an optical router based on the polarization of FW and directionality of SHG signals In order to further demonstrate the usefulness of the strong and directional SHG signals produced from NW devices, we configured an optical router by coupling two CdS NW waveguides. Owing to the anisotropic geometry of NWs, intense SHG is usually generated from the NW under parallel excitation (due to high in-coupling; Fig. 4a ) that radiates orthogonally to the NW ( Fig. 1b and Fig. 5b ). Based on this principle, we investigated two crossed CdS NWs ( Fig. 6a ; NW2 in intimate contact with NW1) by tuning the polarization of the excitation laser at 1,036 nm (corresponding to SHG at 518 nm) focused at the O-junction (where the two NWs meet). At the polarization angle of θ =30° (with respect to the vertical axis in the lab frame, parallel to NW1; Fig. 6a ), the SHG signal generated from NW1 at the O-junction is therefore preferentially coupled into NW2 and transported to its end (point D; Fig. 6b ), which leads to the detected power ~14 times higher at NW2 end (point D) than at NW1 end (point R; Fig. 6e ). If NW1 was excited away from the point O, then the SHG signal would not waveguide along NW1 (as discussed previously and in Supplementary Fig. 11 ) but can be scattered into NW2 benefiting from the directionality of SHG. At θ =90°, NW2 is under parallel excitation and functions as a light source, and the SHG signal (from NW2) is coupled preferentially into NW1 and transported to its end (R-end; Fig. 6d ). Much stronger signal (>3 × ) is achieved at the R-end in comparison with the D-end. Notice that more signal can be coupled into NW2 at θ =30° owing to the end-scattering effect of NW2. Therefore, the contrast ( P D / P R ~14) at θ =30° is higher than that ( P R / P D ~3.5) at θ =90° ( P D ( P R ) is the SHG power at the D- (R-) end). For an intermediate case, for example, θ =70°, the SHG signal can be produced from both the NWs and scattered into the other waveguide ( Fig. 6c ), leading to comparable signal intensities at the two ends (D and R; inset of Fig. 6e ). In order to demonstrate that the router is enabled owing to the unique directionality property of the SHG signals, similar experiments performed on the same system, but exciting only the PL from these wires, exhibited no such routing functionality in response to the change in excitation polarization ( Supplementary Fig. 12 ). 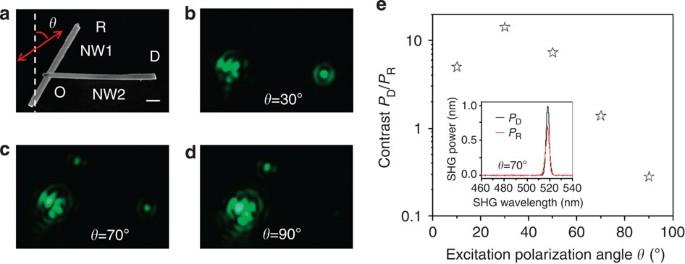Figure 6: Polarization-controlled optical router. (a) Scanning electron microscope image of the nanowire (NW) router showing crossed CdS NWs (NW1 and NW2 in intimate contact). O represents the junction and the laser excitation point, whereas R (or D) stands for the end of NW1 (or NW2). Scale bar, 500 nm. (b) Dark-field image of the crossed NW device when the excitation laser at 1,036 nm is polarized along NW1 (θ=30° with respect to the vertical axis as shown) and focused at the O-junction. (c) Second harmonic generation (SHG) signal observed both at D- and R-ends ifθ=70°. (d) SHG signal routed into NW1 when the excitation polarization is tuned parallel to NW2 (θ=90°). (e) Contrast ratios (PD/PR) of SHG signal power detected at D- and R-ends.PD(orPR) represents the SHG power at D- (or R-) end. Inset: similar SHG signal power at D- and R-ends ifθ=70°. Figure 6: Polarization-controlled optical router. ( a ) Scanning electron microscope image of the nanowire (NW) router showing crossed CdS NWs (NW1 and NW2 in intimate contact). O represents the junction and the laser excitation point, whereas R (or D) stands for the end of NW1 (or NW2). Scale bar, 500 nm. ( b ) Dark-field image of the crossed NW device when the excitation laser at 1,036 nm is polarized along NW1 ( θ =30° with respect to the vertical axis as shown) and focused at the O-junction. ( c ) Second harmonic generation (SHG) signal observed both at D- and R-ends if θ =70°. ( d ) SHG signal routed into NW1 when the excitation polarization is tuned parallel to NW2 ( θ =90°). ( e ) Contrast ratios ( P D / P R ) of SHG signal power detected at D- and R-ends. P D (or P R ) represents the SHG power at D- (or R-) end. Inset: similar SHG signal power at D- and R-ends if θ =70°. Full size image Note that the TM-excited SHG efficiency is ~10 −6 W −1 ( Fig. 1c and Supplementary Fig. 9a ) is much higher than the TE-excited SHG efficiency ~10 −8 W −1 ( Fig. 4c ) for the Ag-coated NWs. Actually in the majority of cases, efficient SHG is usually found to be due to TM-polarized excitation instead of TE-polarized excitation, even if the transverse SPR is excited ( Supplementary Table 3 ). Besides the high in-coupling efficiency under TM excitation, the in-coming FW is concentrated strongly in the nonlinear region (compared with TE-polarized mode) at the resonant wavelength with perfect overlap, which is crucial to optimize the SHG signal. In contrast, the transverse SPR mostly localizes the optical field in the interlayer [27] (SiO 2 , with negligible nonlinear coefficients; Fig. 4d ), which results in poor mode overlap and lower average intensity in the CdS (with very high nonlinear coefficients) region in comparison with TM excitation. Moreover, TM-excited SHG depends on the second-order nonlinear coefficient of d 33 , which is the largest component in the CdS nonlinear tensor and is ~2 times more than d 31 that relates to TE-excited SHG [28] . Note that the measured SHG efficiency enhancement of ~300 obtained for TM excitation (Ag-coated device) in comparison with bare NW ( Fig. 1c ) corresponds to a calculated internal efficiency enhancement of ~2,400 (in- and out-coupling efficiency is ~50% of the bare NW; Supplementary Equation (12) and Supplementary Fig. 4b ). As for the heating of the metal layer, we believe it is not too severe in our devices under the low excitation powers used (0.13–0.9 mW) and also because of the light concentration in the dielectric core (TM 01 ) ( Supplementary Fig. 13 ). Further improvements can be achieved by designing cavities that are also resonant with the SHG signals and also utilizing the higher nonlinearities of CdS excitons [34] . In terms of conversion efficiency, it is important but difficult to make direct and quantitative comparisons between different devices owing to very different material responses and different systems (geometry, size and so on) that will be ultimately used for different applications. Each system based on their size, geometry/form and other properties also has their promises and challenges. For example, a gallium arsenide (GaAs)–WGM microresonator (GaAs–WGM) can produce very strong SHG signal (5 × 10 −2 W −1 ) owing to the large size ( d ~5.2 μm) and high nonlinear coefficient [14] but has a large footprint. Small nanoparticles (<100 nm), for example, BaTiO 3 /Au nanocavity [24] , may find applications in bio-imaging but may not produce strong enough SHG signal power (7.3 × 10 5 GM) to be coupled into other devices such as waveguiding and optical manipulation for on-chip applications. Here, we have designed Ag-coated CdS NWs (~200 nm) for efficient, tunable and directional SHG (3.0 × 10 −6 W −1 or 3.1 × 10 8 GM). Under TM excitation, the lowest-order WGM (TM 01 ) is excited that strongly confines most of the optical mode in the nonlinear region of CdS leading to highly enhanced SHG (>1,000 times stronger in comparison with bare NWs). The strong and directional SHG signals obtained from the device were then coupled into another waveguide to demonstrate coupling between two components, and further utilized to configure an optical router. These device concepts utilizing the enhanced signal strength and unique properties of SHG signals can lead to the development of novel nanophotonic device concepts for on-chip signal processing and other applications [6] . In order to further increase external conversion efficiency, designing special metallic gratings or a bulls-eye aperture [35] to focus or modulate SHG for higher out-coupling efficiency will be beneficial. To achieve similar results while pushing the limits of these devices to smaller sizes, active materials with higher refractive index than CdS (for example, α-ZnS and so on) may be used. These devices with high conversion efficiencies when applied to study other nonlinear processes, such as down-parametric conversion for entangled photon pairs and optical rectification for terahertz radiation will find a wide range of potential applications in biology, physics and chemistry. NW growth and device fabrication Au-catalysed crystalline CdS NWs were grown on silicon substrates at 760 °C in a quartz tube with vapour phase transport of CdS powder by argon (99.999% purity, 100 s.c.c.m.) and then dry-transferred onto a 0.15-mm-thick glass substrate. A 6-nm-thick SiO 2 layer was then deposited by atomic layer deposition (ALD; Cambridge Nanotech) followed by a 200-nm-thick Ag film by electron beam deposition at a low deposition rate of 0.2 Å s −1 for the first 50 nm and 1.0 Å s −1 for the remaining film. After all, the optical measurements were performed, the sample was placed into a Ag etchant, TFS (Transene) for 20 s to remove the Ag deposition completely. Then the diameter of CdS NWs was measured by scanning electron microscopy. Optical measurements Ag-integrated and bare CdS NWs were mounted in a continuous flow optical microscopy cryostat (ST-500, Janis Research) for room and low-temperature measurements ( Supplementary Fig. 2 ). A femtosecond-pulsed Ti:sapphire laser (Chameleon), tuned from 680 to 1,080 nm with ~140 fs pulse width and 80 MHz repletion rate, was focused (spot size ~2 μm) onto individual NWs through the 0.15-mm-thick glass substrate by means of a home-built microscope equipped with a × 60, 0.7 NA objective (Nikon). The average excitation power of ~350 μW (FW) was used to excite SHG from NWs at 950 nm excitation. The SHG signals and two-photon absorption-induced PL were imaged by a cooled charge-coupled device and spectroscopy was performed by a spectrometer (Acton) with a 300 groove per millimetre 500 nm blaze grating and a charge-coupled device detector (Princeton Instruments) with a spectral resolution of 0.1 nm. Numerical calculations and conversion efficiency of SHG signals The SHG signal can be estimated by , where α 2 ω ,ave is the total average absorption of SHG and represents the average intensity of the optical mode excited by FW in the CdS core ( Supplementary Equations (3)–(10) ). By using finite-difference time-domain software (Lumerical), we performed simulations for Ag-coated and bare CdS NWs excited by an external plane wave and obtained the scattering and absorption spectra along with intensity distributions. Then the total average absorption of SHG ( α 2 ω ,ave ) and the average intensity of FW ( I ω ,ave ) was obtained by integrating the electric field over the entire CdS core region. Frequency-dependent refractive index of all materials (Ag, SiO 2 and CdS) was used [36] . The normalized external conversion efficiency is defined as , which is independent of the excitation power and directly reveals the device performance. Here P ω ( P 2 ω ) represents the peak power of FW (SHG). The SHG scattering cross-section, ( I ω , peak intensity), is another commonly used metric to evaluate the conversion efficiency [24] . As to these reported values ( Figs 1c and 4c and Supplementary Fig. 9a ), we have taken into account the system’s collection efficiency of ~0.5% ( Supplementary Discussion ) and excitation efficiency of ~10% (the NW size is much smaller than the excitation spot size). If considering the in-coupling efficiency of FW and out-coupling efficiency of the SHG signal, the internal efficiency can be obtained by . How to cite this article: Ren, M.-L. et al. Enhanced second-harmonic generation from metal-integrated semiconductor nanowires via highly confined whispering gallery modes. Nat. Commun. 5:5432 doi: 10.1038/ncomms6432 (2014).